Low-mass black holes as the remnants of primordial black hole formation Over the last decade we have come to understand that supermassive black holes, with masses of millions to billions of times the mass of the Sun, are very common in the centres of massive galaxies [1] . We would like to understand when and how they formed and grew. We cannot yet watch the first supermassive black holes form. They did so soon after the Big Bang, and light from those distant events is beyond the reach of today’s telescopes. However, we do have two very interesting limits on the formation of the first black holes. The first comes from observations of the most distant known black holes: light is emitted by material falling into the deep gravitational potential of the black hole. These monsters are so bright that they must be powered by at least billion solar mass black holes. They had very little time to grow, as we see them only a few hundred million years after the Big Bang [2] , [3] . Whatever process formed and grew the first supermassive black holes had to be very efficient. At the other extreme, we can study the lowest-mass black holes in galaxy nuclei near to us, the left-over seeds that for some reason never grew to be a billion suns. As we describe below, conditions were best to make supermassive black hole seeds soon after the Big Bang. Therefore, black holes found in small galaxies today, with black hole masses of ∼ 10 4 –10 6 M ⊙ , likely formed early and have not grown significantly since. These black holes have masses between those of ‘stellar-mass’ black holes that form as the end-product of the life of a massive star and supermassive black holes. We will refer to black holes in this mass range as ‘low-mass’ black holes, as they are at the low-mass end of supermassive black holes. If we assume that black holes form in a similar way in all galaxies, then the numbers and masses of black holes in small galaxies today contain clues about the formation of the first black holes [4] . The sheer number of left-overs will indicate how commonly black hole seeds were formed, as well as inform future gravitational wave experiments that expect to see a large number of paired low-mass black holes as they spiral together and coalesce [5] . Studying the energy output from low-mass black holes could tell us whether growing black holes at early times were important in shaping early star formation in the galaxies around them [6] . Unfortunately, low-mass black holes are difficult to find. Because of their low mass, they only have gravitational influence over stars in a very small volume at the galaxy centre. Therefore, we are often forced to wait until material falls into the black hole, when we can detect it indirectly via the radiation that is released. Here I will briefly review different formation paths for the first seed black holes, then describe how astronomers have searched for low-mass black holes. I will discuss the properties of the low-mass black holes that are currently known, and end with hints that a process more exotic than supernova formed primordial seed black holes. To understand the growth of the first supermassive black holes, we first must determine how the black holes form to begin with. Theoretically, there are two possible answers. Either black holes are created as the end-product of stellar evolution, a process that continues to produce stellar-mass black holes today, or the black hole is made directly from the collapse of a gas cloud, which requires the high gas fractions and low metallicities present in the early universe [7] . Once the black hole is formed, it also must grow. There are likely many growth paths, but a rapid mechanism is required to explain the ∼ 10 9 M ⊙ black holes that are observed only hundreds of millions of years after the Big Bang [3] . We first discuss the two formation routes, and then the possible growth mechanisms. Volonteri [7] presents a very cogent and recent review of the leading theories for the formation of the first massive black holes. I will only briefly review the subject for completeness, with an emphasis on the observable consequences at the present day. Stellar-mass black holes form when massive stars run out of fuel at the end of their life. The first black holes may have formed in the same way. The first stars were likely very massive [8] . In order for stars to form, gas clouds need to contract; they are able to cool and shrink by emitting light predominantly in specific element transitions. As there were no elements heavier than He and Li in primordial gas, it was hard for clouds to cool efficiently. As a result, proto-stars grew much larger before their gravitational attraction was strong enough to counteract the internal energy in the gas. In theory, the end-product of these massive first stars will depend on the mass. Stars with masses less than ∼ 100 M ⊙ or more than ∼ 260 M ⊙ will become black holes with masses approaching that of the star [9] . For masses in between, it is thought that pair-instability supernova, in which pair production in the star centre leads to a run-away stellar collapse, will leave no remnant [10] . Of course, the details of early stellar evolution are very difficult to test observationally. There are many uncertain details, such as whether the first stars formed in pairs, and how much mass they lose at late stages of evolution. We will assume the first stars left behind standard ∼ 100 M ⊙ remnants. Alternatively, conditions in the early universe may have allowed gas clouds to collapse directly into black holes [11] . These black holes could form 10 3 –10 5 M ⊙ black holes immediately. Direct collapse requires very-low angular momentum gas that only existed in large quantities soon after the Big Bang. In this scenario, the gas must be kept relatively hot so that it does not fragment into stars. Only a very small fraction of halos will have nearby massive stars to surpress cooling, and only those few will manage to form a black hole [12] . With these two formation paths in mind, the next question is whether the black holes created via either path can grow into the very luminous sources that are observed hundreds of millions of years after the Big Bang. With direct collapse models, even in the halos with low angular momentum content and low molecular hydrogen fraction (and thus inefficient cooling) the gas will likely settle into a disk, and require some sort of instability to condense further [13] . Once sufficiently condensed, the central 10 4 –10 5 M ⊙ of material may very efficiently gain mass as a dense and round ‘quasi-star’ [14] . It is marginally possible for a stellar-mass seed to grow into a billion solar mass black hole in hundreds of millions of years, but only if the black hole manages to grow continuously at the maximal allowed rate. Above the so-called ‘Eddington’ limit, gravity pulling in can no longer balance radiation pushing outward. In practice, it is difficult for black holes to grow continuously at their Eddington limit, as the emission from accretion will heat the gas around the black hole and slow down subsequent accretion [15] . One way to speed up the growth of black holes created via stellar death is to merge many smaller seeds into a more massive seed [16] . Dense clusters of stars contain many small seeds that may sink to the centre of the cluster and merge to form a more massive seed with M BH ≈10 4 M ⊙ that can then grow further into a supermassive black hole [17] . Similarly, stars may merge first, forming a supermassive star and then create a more massive seed [18] , [19] . Observational consequences These different formation scenarios are only interesting if they predict differences in observations of the real universe. Eventually, perhaps with the James Webb Space Telescope, successor to the Hubble Space Telescope, we will detect the earliest growing black hole seeds [8] . In the meantime, we can look for clues in how black holes inhabit galaxies today. Just looking at supermassive black holes in massive galaxies provides few insights, because all memory of their humble beginnings has been erased through the accretion of gas and smaller black holes. However, if we focus on the ‘left-over’ seeds in small galaxies (those with stellar masses M gal <10 10 M ⊙ ), the black holes that never grew, we get a more direct view of the original seed population [4] . Volonteri et al . [20] construct models of dark matter halos merging and growing from the early universe to the present day. They put seed black holes into the halos using different prescriptions depending on how the seeds were formed ( Fig. 1 ). Then, they watch the black holes evolve along with the halos. There are still many uncertainties associated with these models. For instance, as black holes merge, they emit gravitational radiation. In general, the gravitational radiation will have a preferential direction. When the black holes finally merge, the remnant black hole will receive a kick from the gravitational radiation that may, in extreme cases, send the black hole out of the galaxy completely, through a process called gravitational ‘recoil’ [21] . As it is theoretically uncertain how effective gravitational radiation will be at ejecting black holes, there is additional uncertainty added to the models. Also, the models assume seeds are formed either via direct collapse or via star death, when in reality there is likely a mixture. 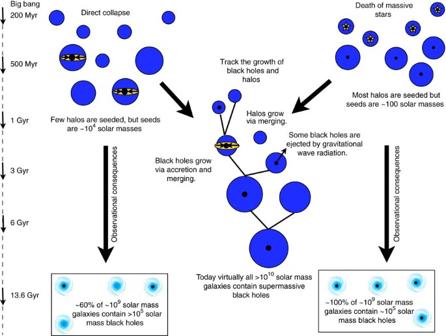Figure 1: Evolution of seed black holes. Schematic of the evolution of seed black holes assuming two different formation mechanisms (the death of the first generation of massive stars versus the direct collapse of gas into a black hole). Dark matter halos and the galaxies in them grow through merging. Black holes grow both via merging and by accreting gas. One additional complication is that after merging, gravitational radiation ‘recoil’ (see text for details) may send the black hole out of the galaxy. At present, we can distinguish between the two scenarios based on the fraction of small galaxies that contain massive black holes (we call this the ‘occupation fraction’). Figure 1: Evolution of seed black holes. Schematic of the evolution of seed black holes assuming two different formation mechanisms (the death of the first generation of massive stars versus the direct collapse of gas into a black hole). Dark matter halos and the galaxies in them grow through merging. Black holes grow both via merging and by accreting gas. One additional complication is that after merging, gravitational radiation ‘recoil’ (see text for details) may send the black hole out of the galaxy. At present, we can distinguish between the two scenarios based on the fraction of small galaxies that contain massive black holes (we call this the ‘occupation fraction’). Full size image Given these uncertainties, we focus on the qualitative aspects of the models. They predict a higher fraction of low-mass galaxies to contain nuclear black holes if seeds are created via stellar deaths (see ref. 20 and the purple solid and green dashed lines, respectively, in Fig. 2 ). We are trying to measure the fraction of galaxies that contain low-mass black holes, particularly in host galaxies with M gal <10 10 M ⊙ . As I will show, this work is still in progress. 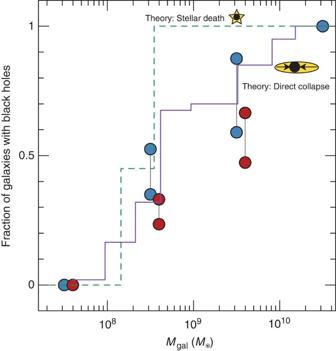Figure 2: The Occupation Fraction. We show the expected fraction of galaxies withMgal≲1010M⊙that contain black holes withMBH≳3 × 105M⊙, based on the models of ref.20, as presented in ref.7, for high efficiency massive seed formation (solid purple line), as well as stellar deaths (green dashed line). Using data from the literature, the large circles show the fraction of galaxies containing black holes greater than 106M⊙(lower points) and greater than 3 × 105M⊙(higher points) based on Desrocheset al.52(blue) and Galloet al.50(red). The difference between the two roughly represents the systematic errors in the methods. See text for details. Although the uncertainties are very large, we find tentative evidence in support of the efficient massive seed models (purple solid line). Figure 2: The Occupation Fraction. We show the expected fraction of galaxies with M gal ≲ 10 10 M ⊙ that contain black holes with M BH ≳ 3 × 10 5 M ⊙ , based on the models of ref. 20 , as presented in ref. 7 , for high efficiency massive seed formation (solid purple line), as well as stellar deaths (green dashed line). Using data from the literature, the large circles show the fraction of galaxies containing black holes greater than 10 6 M ⊙ (lower points) and greater than 3 × 10 5 M ⊙ (higher points) based on Desroches et al . [52] (blue) and Gallo et al . [50] (red). The difference between the two roughly represents the systematic errors in the methods. See text for details. Although the uncertainties are very large, we find tentative evidence in support of the efficient massive seed models (purple solid line). Full size image Astrophysical supermassive black holes were first discovered as ‘QSOs’—quasi-stellar objects with very-high intrinsic luminosities and very small sizes [22] . By the late 1970s there was compelling evidence that quasi-stellar objects are powered by accretion onto a supermassive black hole. They were called ‘active galactic nuclei’ because they were shining via the energy released as material falls into (or is accreted by) the central supermassive black hole [23] . The existence of real supermassive black holes, with masses of hundreds of millions of times the mass of the Sun became commonly accepted, but it was far less clear whether these monsters represented a rare and long-lived phenomenon, or whether all galaxies contained supermassive black holes with short-lived bright episodes. Twenty years later we finally learned that supermassive black holes are common. In fact, we believe that most massive galaxies contain a central supermassive black hole. The evidence came from both stellar dynamics and accretion ( Box 1 ). A survey by Ho et al . [24] searched the centres of nearby, ‘normal’ galaxies for subtle evidence that trace amounts of gas was falling into a central black hole. Amazingly enough, most ( ∼ 70%) massive galaxies showed clear signs of accretion onto a supermassive black hole (see review in ref. 25 ). At the same time, stellar dynamical work was providing increasing evidence that every bulge-dominated galaxy harbours a supermassive black hole [1] . It became clear that black holes were preferentially associated with galaxy bulges. (Bulges are ellipsoidal in shape and comprises mostly old stars that move on random orbits through the galaxy. In contrast, disks are flat components of galaxies, where stars all orbit the galaxy on coplanar circular paths. Disks contain gas and ongoing star formation. If a bulge component contains no disk, we call it an elliptical galaxy). Furthermore, the ratio of black hole to bulge mass was apparently constant to within a factor of two to three [26] . Unfortunately, understanding the black hole population becomes increasingly challenging as one considers lower and lower-mass galaxies. Low-mass galaxies typically contain more cold gas, more dust and higher levels of ongoing star formation. The dust obscures emission from accretion, while the star formation masks it. Furthermore, if the correlation between black hole mass and bulge mass applies, the black holes in smaller galaxies are less massive, which makes their emission weaker. Dynamical evidence for black holes in low-mass galaxies For the handful of low-mass galaxies nearest to us, it is possible to search for the gravitational signature of a central black hole. In stark contrast to bulge-dominated galaxies, these nearby small galaxies show no evidence for a central massive black hole, with an upper limit of 1,500 M ⊙ for the galaxy M33 (ref. 27 ) and of 10 4 M ⊙ for NGC 205 (ref. 28 ). Lora et al . [29] and Jardel and Gebhardt [30] find that the black hole masses of two very-low-mass dwarf galaxies in our local neighbourhood cannot be larger than ≲ 10 4 M ⊙ . While most massive, bulge-dominated galaxies contain black holes (an ‘occupation fraction’ close to unity), clearly the occupation fraction drops in low-mass galaxies without bulges. Do 50% of dwarf galaxies contain black holes or only 1%? And how does that fraction change with the mass of the galaxy? I adopt a transition mass of 10 10 M ⊙ , based on the findings from the Sloan Digital Sky Survey (SDSS) that active galaxies become rare below this stellar mass [31] . Apart from M33 and NGC 205, there are very few galaxies near enough to place interesting limits on the presence or absence of a black hole based on the motions of stars or gas at the galaxy centre ( Box 1 ). Barth et al . [32] studied the nuclear kinematics of the bulgeless galaxy NGC 3621. This galaxy also shows some evidence for accretion ( Box 1 ). They place a very conservative upper limit of 3 × 10 6 M ⊙ on the mass of a central massive black hole, which would be improved by better measurements of the stellar ages in the star cluster surrounding the black hole. Seth et al . [33] used the motions of a gas disk in the centre of the small S0 galaxy NGC 404 to find a likely black hole mass of ∼ 5 × 10 5 M ⊙ . Neumayer and Walcher [34] find upper limits of ∼ 10 6 M ⊙ for nine bulgeless spirals, confirming that such galaxies contain low-mass black holes if they contain a central black hole at all. Bulgeless galaxies with active nuclei M33 taught us that not all low-mass galaxies contain central supermassive black holes. The galaxy NGC 4395, a galaxy very similar in mass and shape to M33, shows that some low-mass galaxies do contain nuclear black holes [35] . Like M33, NGC 4395 is small and bulgeless. Unlike M33, NGC 4395 contains unambiguous evidence for a central massive black hole ( Box 1 ), including extremely rapid variability in the X-rays [36] and a radio jet [37] . While we do not know precisely, the black hole mass is likely 10 4 –10 5 M ⊙ ( [38] , [39] , [40] ). NGC 4395 highlights the utility of using nuclear activity as a fingerprint of low-mass black holes when their gravitational signature is undetectable. In 2004, Aaron Barth reobserved the forgotten active galaxy POX 52 ( [41] , [42] ), which has a near-identical optical spectrum to NGC 4395. POX 52 also appears to contain a ∼ 10 5 M ⊙ black hole. NGC 4395 went from being an unexplained oddball to the first example of a class of objects, with POX 52 being the second example. But are there more? Greene and Ho [43] were inspired to perform the first large systematic search for this new class of ‘low-mass’ accreting black holes. In 2003, the SDSS [44] had just started to provide pictures and spectra of objects over one-quarter of the sky, exactly what was needed to search for the rare and elusive low-mass black holes. Greene and Ho [43] went through hundreds of thousands of galaxy spectra to pick out the accreting black holes with fast-moving gas at their centres ( Box 1 ). They then picked out the ∼ 200 systems with masses <10 6 M ⊙ ( [43] , [45] ). Greene and Ho chose this mass because it is similar to the mass of the black hole at our galaxy centre, and serves as the anecdotal low-mass cutoff of supermassive black holes. Dong et al . [46] also searched through the SDSS for low-mass black holes with similar criteria, increasing the total sample by ∼ 30%. Subsequent searches of the SDSS have adopted different approaches. While looking for galaxies with pristine, metal-free gas, Izotov and Thuan [47] present evidence for accreting black holes in four vigorously star-forming galaxies, again based on the detection of fast-moving gas that is most likely orbiting a black hole with M BH ∼ 10 4 –10 6 M ⊙ ( Box 1 ). In contrast, a number of groups are now first selecting low-mass galaxies, and then searching for signatures of accretion (ref. 48 ). Multiwavelength searches Searches for low-mass black holes using the SDSS were an important first step, and allowed us to comb through hundreds of thousands of galaxies. However, they are fundamentally limited in two ways. First, in galaxy nuclei with ongoing star formation, dust obscuration and emission from star formation hides the evidence of nuclear activity. Second, the SDSS takes spectra of a biased sample of relatively bright galaxies, which makes it very difficult to calculate a meaningful occupation fraction [49] . An obvious way to circumvent these biases, and complement the original optical searches, is to use other wavebands. X-rays, for instance ( Box 1 ), are such high-energy photons that they can only be hidden by very large quantities of gas. Radio and mid-infrared wavelengths are also relatively unaffected by dust absorption. On the other hand, multiwavelength searches to date have been restricted to small samples. The fraction of low-mass ( M gal <10 10 M ⊙ ) galaxies with X-ray emission coming from the nucleus has been studied both as a function of stellar mass [50] , [51] and galaxies comprising old stars morphology [52] , [53] . The former studies focused on galaxies comprises old stars, while the latter focused on star-forming galaxies. Less than 20% of non-star-forming galaxies with M gal <10 10 M ⊙ have nuclear X-ray sources with L X ≳ 2.5 × 10 38 erg s −1 , while in star-forming galaxies of similar mass, ∼ 25% of galaxies contain X-ray nuclei above the same luminosity. The difference in detection rate is likely due to a lack of gas to consume in the red galaxies. Below, I will use these detection fractions to estimate the occupation fraction in galaxies with M gal <10 10 M ⊙ . The X-ray luminosities probed here are very low. If a 10 5 M ⊙ black hole has very little to accrete, it will only shine very weakly, in this case with an X-ray luminosity as low as L X ≲ 10 38 erg s −1 . However, stellar-mass black holes can sometimes shine with this luminosity as well, although they are not very common; the best guess is that ∼ 10% of the sources are actually powered by 10 M ⊙ black holes while the rest are powered by ∼ 10 5 M ⊙ black holes [50] . However, as we look at less and less luminous X-ray sources, more and more of them will be powered by stellar-mass black holes. A luminosity of L X ≲ 10 37 erg s −1 is a typical luminosity for a radiating stellar-mass black hole and so at this luminosity nearly all detected sources will be stellar-mass black holes. Owing to confusion about the nature of the detected objects, we are reaching the limit of what X-ray searches alone can tell us about the demographics of low-mass black holes. It is possible that including X-ray variability information will also help weed out the stellar-mass black holes [54] . The high-ionization [Ne V] line, detected in mid-infrared spectroscopy, is a reliable indicator of active galactic nuclei activity since starlight likely cannot excite this transition [55] . Satyapal et al . [56] , [57] focus on galaxies with little to no bulge component. In galaxies with very small bulges, they find a detection fraction similar to the X-ray studies ( ∼ 20%; see also ref. 58 ) but in galaxies with no bulge whatsoever, their detection fraction drops nearly to zero [58] (one galaxy out of 18 contains a [Ne V] detection). While the precipitous decline of detected bulgeless galaxies provides evidence for a dramatic decline in the occupation fraction of bulgeless galaxies, it is worth noting that the observations of the latter galaxies were not as sensitive. Further progress requires observations at multiple wavelengths. For example, Reines et al . [59] identified a likely 10 5 –10 6 M ⊙ black hole in the centre of the low-mass star-forming galaxy Henize 2–10. Radio or X-ray emission alone would have been unconvincing, as either could easily be explained by processes relating to star formation. However, the spatial coincidence of the radio and X-ray source, their relative brightness and their distance from clusters of forming stars make a compelling case for a low-mass black hole in this galaxy. A larger sample of galaxies similar to Henize 2–10 also appear to have accreting black holes in some cases. Again, it is the combination of X-ray and radio detections that argues for black holes in these galaxies [60] , [61] . Box 1: Finding supermassive black holes. Direct detection with stellar dynamics The most direct way to demonstrate that a supermassive black hole exists at the centre of a galaxy is to look for its signature from the motions of gas or stars at the galactic nucleus. Just like planets going around the Sun, the laws of gravity can translate the average velocities of stars around the black hole into a mass. At the centre of our own Milky Way galaxy, researchers have charted the motions of individual stars whipping around the galaxy centre for over two decades. Their motions provide unambiguous evidence for a 4 × 10 6 M ⊙ black hole [83] , [84] . In other galaxies, we cannot study individual stars but we can still see the black hole signature in the average star motions near the galaxy centre. Stars move much faster on average if there is a black hole at the centre of the galaxy than if there isn't. The more massive the black hole, the faster the average motions of the stars. As the black hole comprises only a fraction of a per cent of the total mass of the galaxy, only stars or gas very near the galaxy centre can feel its gravitational attraction. Detecting these fast-moving stars requires either the high spatial resolution of the Hubble Space Telescope or adaptive optics from the ground. Orbiting gas clouds can also be used to weigh the black hole, using very similar principles [85] , [86] . It is only possible to detect the gravity of big black holes that are in relatively nearby galaxies. Comparing the top- and bottom-left panels, the signal from the gravity of the black hole is strongly concentrated towards the galactic centre. When the galaxy is furtheraway, the motions of stars near the black hole are blurred together with more distant stars that don’t feel the black holes gravity, making its influence imperceptible. Similarly, as the black hole mass gets smaller, high-velocity stars become harder to detect. To study low-mass black holes, we must generally wait until matter falls into the black hole and forms an accretion disk, which we can detect. Detecting accretion onto black holes Occasionally, gas makes its way into the galaxy nucleus and into the black hole. However, it must dissipate its energy and angular momentum to fall into the deep gravitational potential of the black hole. Nature uses accretion disks to funnel matter into black holes. Accretion disks radiate most of their energy in the ultraviolet. While we cannot see the peak of the radiation from the accretion disk, we recognize the following signatures of an accreting black hole listed below (see schematic in top right panel). First, we see X-ray emission at the galaxy nucleus. High-energy interactions between photons and electrons form an X-ray corona above the accretion disk. As the corona region is very compact, the light signals propagate from one side of the corona to the other rapidly, enabling variability on short timescales. X-rays from the accreting black hole are much more luminous than those from other processes in the galaxy. Sometimes accretion is accompanied by jets of accelerated particles that emit radio waves. Jet emission often accompanies accretion disks, although the exact mechanisms responsible for launching these jets are not fully understood. Outside the accretion disk, gas orbiting the black hole emits spectral line transitions. For instance, hydrogen atoms emit optical light when electrons fall into the second energy level. Intrinsically, light from electron transitions is emitted at a specific frequency, but because the gas is moving towards and away from us, the frequency we observe is shifted to the blue or the red via the Doppler shift. The faster the gas moves, the wider is the range of velocities that we observe in line emission, and hence a broader line arises. The fast-moving gas orbiting close to the black hole but outside the accretion disk is called the ‘broad-line’ region because of the high observed velocities (bottom right panel). The gas in the galaxy on larger scales is also illuminated by emission from the accretion disk. As the accretion disk emits strongly in the ultraviolet and X-rays, the gas is excited to a wide range of temperatures. Gas excited by accretion shows specific fingerprints in the ratios of different atomic transitions. Using accretion to determine black hole mass If we cannot determine a black hole mass directly using star or gas motion, we approximate it by observing the motions of gas clouds in the broad-line region: the faster the gas moves on average, the wider the range of observed velocities, and the more massive the black hole. Distance from the black hole matters as well. By analogy with our solar system, Pluto is further from the Sun and thus moves much more slowly around the Sun than Earth does. In the case of the gas clouds, it is challenging to determine their distances from the black hole. In some cases the time delay in variable emission from the accretion disk itself, and from the broad-line region further away, provides a size scale for the emission region. The distance is just the delay time times the speed of light. Using this technique, the mass of the black hole in NGC 4395 is found to be M BH ≈10 5 M ⊙ ( [38] , [39] ). Measuring these time delays is very time consuming. Usually, we do not measure the broad-line region size directly. Instead, we use a correlation between the luminosity of the black hole and the broad-line region size to estimate a radius for the broad-line region gas. In addition to measuring the fraction of low-mass galaxies that contain black holes, it is of interest to determine whether black holes with lower-mass emit a different spectrum than more massive accreting black holes. For instance, one naively expects that the accretion disk will get physically smaller and thus hotter as the black hole mass decreases. In turn, gas in the vicinity of the black hole will be heated by more energetic photons. Predictions of the impact of low-mass black holes on the gas conditions in the early Universe require empirical measurements of the radiation from low-mass black holes. In practice, as accretion disk emission around supermassive black holes peaks in the ultraviolet, it is difficult to unambiguously measure changes in the disk temperature with mass [62] . We have measured a few intriguing properties of the radiation from low-mass black holes, although thus far we have studied only the most luminous of them. First, they appear to have a very-low incidence of jet activity [63] . Second, we see indirect evidence that they have hotter accretion disks than their more massive cousins [64] , [65] , [66] , as expected from basic disk models [67] . As the accretion disk gets hotter, its impact on the surrounding gas will grow. Thus, growing black holes may well impact the formation of the first stars and galaxies [6] . Accretion onto a central black hole has been found in low-mass galaxies of all shapes and with all levels of ongoing star formation. Miller et al . [51] have found accreting black holes in galaxies comprised predominantly of old stars, while Izotov and Thuan [47] , Reines et al . [59] , and Jia et al . [60] have reported evidence of accreting black holes in vigorously star-forming galaxies. Some host galaxies are round [41] , while others are pure disks [40] . We display the variety of host galaxy morphologies in Fig. 3 . 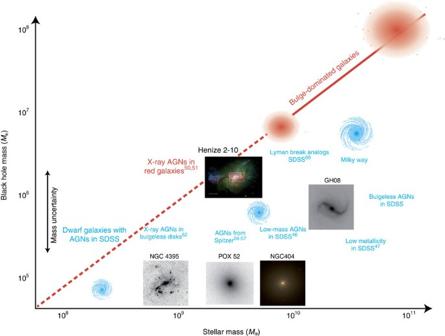Figure 3: Galaxy mass versus black hole mass. The ratio of black hole mass to bulge mass is constant for bulge-dominated galaxies, as shown by the solid red line in the upper right81. To guide the eye, this relationship is extrapolated down to lower black hole masses by the dotted red line. However, in disk-dominated galaxies, particularly at low mass, there is no tight correlation betweenMBHand properties of the galaxy. We illustrate the wide range of galaxy types hosting low-mass black holes, roughly placed in accordance with galaxy and black hole mass. However, note that only NGC 404 (ref.33) has a direct dynamical black hole mass measurement. In all other cases, the black hole masses are very approximate, as illustrated by the error bar to the left. Blue denotes galaxies with ongoing star formation, while red denotes those galaxies with little ongoing star formation. See ref.43for information on the discovery of GH08. Image of NGC 4395 (ref.40) taken from the NASA/IPAC Extragalactic Database. Image of Henize 2–10 from ref.59. Image of POX 52 from ref.82, reproduced with permission from the American Astronomical Society (AAS). Image of NGC 404 courtesy of NASA/STScI. Figure 3: Galaxy mass versus black hole mass. The ratio of black hole mass to bulge mass is constant for bulge-dominated galaxies, as shown by the solid red line in the upper right [81] . To guide the eye, this relationship is extrapolated down to lower black hole masses by the dotted red line. However, in disk-dominated galaxies, particularly at low mass, there is no tight correlation between M BH and properties of the galaxy. We illustrate the wide range of galaxy types hosting low-mass black holes, roughly placed in accordance with galaxy and black hole mass. However, note that only NGC 404 (ref. 33 ) has a direct dynamical black hole mass measurement. In all other cases, the black hole masses are very approximate, as illustrated by the error bar to the left. Blue denotes galaxies with ongoing star formation, while red denotes those galaxies with little ongoing star formation. See ref. 43 for information on the discovery of GH08. Image of NGC 4395 (ref. 40 ) taken from the NASA/IPAC Extragalactic Database. Image of Henize 2–10 from ref. 59 . Image of POX 52 from ref. 82 , reproduced with permission from the American Astronomical Society (AAS). Image of NGC 404 courtesy of NASA/STScI. Full size image Supermassive black holes in bulge-dominated galaxies obey remarkably tight correlations between black hole mass and the properties of the host galaxy. For a long time it was simply unknown whether the correlations seen for bulges apply to disk-dominated galaxies; dynamical black hole mass measurements in disk galaxies are severely compromised by the presence of dust and young stellar populations. Early on, based on very indirect arguments, we saw evidence that the relationship between black holes and galaxies extended to low-mass and even bulgeless systems [68] . However, as the number of available dynamical black hole masses in disk galaxies grows, it becomes increasingly clear that disk-dominated galaxies do not obey tight scaling relations with the central supermassive black hole [69] , [70] , [71] . Apparently the physical process that builds galaxy bulges (the merging of galaxies, we think), is also instrumental in growing black holes and establishing the scaling relations between black holes and bulges [72] . Let us now determine whether existing observations of low-mass black holes favour a particular formation route for primordial seed black holes. I want to estimate the fraction of galaxies containing black holes as a function of galaxy mass: the occupation fraction. Based on previous work, we assume that all galaxies with stellar-mass M gal >10 10 M ⊙ contain black holes. To study the occupation fraction in lower-mass galaxies, I will use the two X-ray studies discussed above from Desroches and Ho [52] and Gallo et al . [50] , combined with that of Miller et al . [51] Note that existing optical studies, while they include a larger number of objects, cannot be used for measuring occupation fractions because of their bias towards luminous host galaxies. While the samples with X-ray measurements are smaller, they should be less biased. As we are using accretion to discover black holes (via X-ray emission), we will not detect all black holes. For instance, we may detect X-rays from 10% of galaxies with M gal =10 11 M ⊙ , while they all contain supermassive black holes. If we then detect X-rays from 1% of galaxies with M gal =10 8 M ⊙ , we can conclude that only 10% of M gal =10 8 M ⊙ contain black holes. We are making an assumption that the fraction of active black holes is always the same (in my example, 10%), independent of the galaxy or the black hole mass. This is a strong assumption that we must make in order to proceed, but in detail it is probably incorrect. For instance, galaxies with less gas may be less likely to harbour an active black hole. For each X-ray sample we need a comparison sample of more massive galaxies with similar X-ray observations. The Gallo et al . [50] sample spans a wide range in stellar mass, so the comparison sample of bulges is built in. As a complementary sample of more massive disk galaxies to compare with the Desroches sample [52] , I take the archival X-ray survey of Zhang et al . [73] The only additional complication is that lower-mass black holes are intrinsically more difficult to detect. Recall that every black hole has a maximum luminosity, where the force of gravity just balances the outward force from radiation (the Eddington limit). A black hole that is ten times more massive will have a limiting luminosity that is ten times higher, and will be ten times easier to detect at a given distance. To make the selection fair, I remove the faintest big black holes from the counting, as we would never find the comparably faint low-mass black holes. In other words, I only count black holes that are all radiating above a fixed fraction of their maximum luminosity. Specifically, I only count black holes radiating above one ten-thousandth of their Eddington limit. This limit allows me to have a decent sample of objects in the massive comparison sample and also to consider limits on the presence of black holes with masses M BH ≳ 3 × 10 5 M ⊙ (as set by the sensitivity of existing X-ray surveys). In most cases I do not have direct measurements of black hole mass. Galaxies with M gal >10 10 M ⊙ are assigned a black hole mass based on the correlation between galaxy mass and black hole mass. Galaxies with M gal <10 10 M ⊙ are just assigned a black hole with a mass between 3 × 10 5 and 10 6 M ⊙ . To calculate uniform stellar masses for all galaxies in both samples, I follow Gallo et al . [50] and use correlations between galaxy B – V colour and the mass-to-light ratio of the stars from Bell et al . [74] I use these mass estimates to calculate the limiting luminosity, and then decide whether or not to include the black hole in the sample. I then compare the number of accreting black holes in galaxies with M gal >10 10 M ⊙ to those with lower mass. The results are shown in Fig. 2 . The Desroches and Ho limits [52] are shown in blue, while the Gallo points [50] are shown in red, for M BH =10 6 M ⊙ (lower) and M BH =3 × 10 5 M ⊙ black holes (upper). The expectations from theory for seeds created via stellar death (green dashed) and direct collapse (solid purple) are shown as well. Obviously, the limits are not yet good enough to say anything definitive, but tentatively the data seem to prefer massive seed models. It is clear that the two samples yield different results. The differences between the two are a good indication of our uncertainties. The uncertainties are close to a factor of two for these limited black hole masses, while if I considered even smaller black holes, the observations would be consistent with almost any occupation fraction. Improving these limits will require a multi-pronged approach. As argued above, the utility of X-ray surveys alone are limited due to confusion from stellar-mass black holes, although X-ray surveys that stare at the same part of the sky for a very long time may be able to find accreting black holes in more distant low-mass galaxies. At the same time, combining sensitive radio and X-ray surveys may yield interesting new constraints on black holes with much lower luminosity. How can we make progress on determining the space density of the lowest-mass black holes? At the moment, we are limited by the largest distances that we can probe in unbiased samples. Optical spectroscopic surveys such as the SDSS have yielded large samples, but with selection biases that are difficult to quantify. Searches in other wavebands, while cleaner in terms of selection effects, reach limited distances and thus contain small numbers of objects. I see multiple paths forward (see Box 2 for an alternative direction). The first is to look harder for black holes in local galaxies. We are reaching a fundamental limit in using X-rays, as stellar-mass black holes will dominate the emission in surveys that push an order of magnitude deeper [50] . On the other hand, the increased sensitivity of radio telescopes (particularly the Jansky Very Large Array) open the possibility of a combined radio and X-ray survey. While on an object-by-object basis there still may be complications [75] , the combination of a radio and X-ray source will be compelling evidence for a low-mass black hole. Likewise, we may be able to rely on variability (both in the X-ray and in the optical) in the future [54] . The second path is to try to find more accreting black holes in small galaxies by searching over larger distances rather than by looking for intrinsically less luminous sources. Very sensitive X-ray surveys [76] should allow such experiments, while the newly refurbished Jansky Very Large Array could perform a very sensitive search using radio wavelengths. We also need better measurements of the fraction of more massive galaxies containing accreting black holes, as our comparison sample [58] . Third, even if a black hole is completely inactive, and thus undetectable by most of the methods discussed here, every once in a long while a star will wander too close to the event horizon of the black hole and get disrupted. Many tidal disruption candidates have been observed (for example, refs 77 , 78 ), likely of stars falling into ∼ 10 6 –10 7 M ⊙ black holes. As tidal disruption events are rare, with at most one every 10 5 years per galaxy expected [79] , we must monitor many galaxies every year to detect tidal disruption events. Ongoing and upcoming projects are designed to look at the same part of the sky again and again over years; with these surveys we can hope to detect many tidal disruptions per year, even around low-mass black holes [80] . Eventually, as the surveys progress, we may be able to use the detection rate of tidal disruptions in small galaxies as an indicator of the occupation fraction. There are many surprises still to come. Box 2: Off-nuclear black holes. In this review, I have focused on black holes found at galaxy centres. However, I will highlight two other very interesting locations that may harbour hitherto unknown low-mass black hole populations: the centres of dense stellar clusters and the outer parts of galaxies. Another route to seed black hole growth may occur if the original seed is formed in the centre of a dense cluster of stars. The black hole might grow to 10 4 –10 6 M ⊙ by accreting smaller black holes [87] . Then we may expect to find ∼ 10 4 M ⊙ black holes at the centres of globular clusters. These dense clusters of stars comprise some of the oldest stellar systems in the universe. Despite many searches for black holes in stellar clusters, both using dynamical techniques [88] and looking for signatures of accretion [89] , there is not yet definitive evidence for black holes in globular clusters. There is one exception. The most massive globular clusters, we believe, were formed not as isolated clusters of stars but rather as the nuclei of galaxies that were then torn to shreds as they were eaten by larger galaxies. These most massive clusters also tend to show a wider range of stellar ages and chemical compositions than is seen in typical globular clusters, suggesting that they were formed gradually rather than as a single unit. The three prominent stripped galaxy candidates that are in our own local neighbourhood all show dynamical evidence for a central 10 4 M ⊙ black hole [90] , [91] , [92] , although the detections are still controversial [93] . Radiation from these putative black holes has not yet been detected [75] , [94] . Another suggestive line of evidence for black holes in the centres of star clusters come from the intriguing ‘ultra-luminous’ X-ray sources (ULXs). As the name implies, these targets have very-high X-ray luminosities, so high that they exceed the maximum (Eddington) luminosity for a stellar-mass black hole. An easy way to explain the high luminosities is to power these X-ray sources with intermediate-mass black holes with masses of 100–10,000 M ⊙ . The evidence is not ironclad, however, as it is possible to reproduce the properties of ULXs with stellar-mass black holes in all but a few extreme cases (for example, Socrates and Davis [95] ). Unfortunately, determining the masses of black holes that power ULXs has proven challenging. There is a spectacular ULX that deserves mention. ESO 243-49 HLX-1 has an X-ray luminosity greater than 10 42 erg s −1 , the Eddington luminosity for a 10 5 M ⊙ black hole [96] . The X-ray source is found offset from the main body of the galaxy ESO 243-49, but at the same distance as the galaxy [97] . HLX-1 is likely embedded in a stellar cluster with M gal ≈10 6 M ⊙ ( [98] ), perhaps the remnant of a galaxy that was eaten by ESO 243-49 in the past. ESO 243-49 HLX-1 is an intriguing source, but so far no other sources like it are known. It is quite possible that many intermediate-mass black holes may reside outside of galaxy nuclei. As galaxies merge, they acquire black holes, as well as stars. Many of these black holes may never reach the galaxy centre, but reside in galaxy halos [99] , where they would be very difficult to find. At higher redshift, the number of infalling accreting black holes is high [100] , while at low redshift, systems like ESO 243-49 HLX-1 appear to be rare. How to cite this article: Greene, J. E. Low-mass black holes as the remnants of primordial black hole formation. Nat. Commun. 3:1304 doi: 10.1038/ncomms2314 (2012).